Evolution of hidden localized flow during glass-to-liquid transition in metallic glass For glasses, the structural origin of their flow phenomena, such as elastic and plastic deformations especially the microscopic hidden flow before yield and glass-to-liquid transition (GLT), is unclear yet due to the lack of structural information. Here we investigate the evolution of the microscopic localized flow during GLT in a prototypical metallic glass combining with dynamical mechanical relaxations, temperature-dependent tensile experiments and stress relaxation spectra. We show that the unstable and high mobility nano-scale liquid-like regions acting as flow units persist in the glass and can be activated by either temperature or external stress. The activation of such flow units is initially reversible and correlated with β-relaxation. As the proportion of the flow units reaches a critical percolation value, a mechanical brittle-to-ductile transition or macroscopic GLT happens. A comprehensive picture on the hidden flow as well as its correlation with deformation maps and relaxation spectrum is proposed. Normal liquids can flow instantaneously on mechanical agitation while the flow in a viscous or a solid glass appears to occur only when the external stress reaches a critical value of yield stress or the temperature reaches the glass transition temperature T g (refs 1 , 2 , 3 ). Apart from the stress-induced instantaneous flow of yield, recent experiments and numerical simulations also demonstrated that a glass subject to stress, which is much smaller than its normal yield strength, can also undergo an extreme slow flowing, which is hard to be detected within a short period of time due to the slowness [4] , [5] , [6] , [7] . On the other hand, the universal nano-scaled localized β-relaxation in metallic glassy state has been observed before the large-scale α-relaxation, which has been demonstrated to be related to the nano-scaled microscopic hidden flowing phenomenon [8] , [9] , [10] , [11] , [12] . However, the structural origin of the flowing phenomena in metallic glasses (MGs) such as the slow flowing and instantaneous flow of yield, elastic and plastic deformations, the transition between the β-relaxation to the α-relaxation and glass to supercooled liquid transition are not clear yet due to the lack of clear structural information. Due to the glassy substances are usually used below their T g (refs 13 , 14 , 15 ), the understanding of its flowing phenomena and the structural evolution path during glass-to-liquid transition, and especially its correlation with their mechanical behaviours, are of crucial practical importance. From the theoretical perspective, a general understanding of the structural origin and evolution of the flow behaviour in the extreme viscous glassy solids could be helpful for the clarification of the intriguing dilemmas of glass nature. Intensive work concentrated on the liquid-to-glass transition or slow down process [16] , [17] . However, the reverse glass-to-liquid transition (GLT) process as well as its structural origin has not been paid enough attention. The characteristic changes and their intrinsic correlations with GLT process are still far from being thoroughly studied. Recent studies on the atomic-scale glassy structure have revealed the existence of liquid-like sites in glassy state [4] , [18] , [19] , which are presumed to be responsible for the viscoelastic flow behaviour in glasses [20] , [21] , [22] . Meanwhile, the studies on glasses have demonstrated that the β-relaxation is identified to play an essential role in the GLT process [2] , [8] , [9] , [11] , [23] , and the β-relaxation has comparable activation energy with that of the deformation unit and strongly correlated with mechanical brittle-to-ductile transition in MGs [20] , [21] , [24] , [25] , [26] , indicating that the β-relaxation is closely related to the initiation and evolution of the localized liquid-like deformation units or flow units in MGs [27] , [28] , [29] , [30] . Yet, the fraction and evolution of these liquid-like zones, leading to the flow phenomena such as elastic and plastic deformations and GLT, are still speculative due to the lack of abundant experimental evidence, and the intrinsic correlations between such deformation transition, relaxation mode and structural characteristics changes during GLT are still poorly understood. In this paper, we apply stress relaxation method covering a wide temperature range and dynamical mechanical analysis, which can detect the β-relaxation to investigate the evolution process of GLT in MG, which can be simply treated as random stacking of hard spheres [31] , [32] , [33] . A La 60 Ni 15 Al 25 MG, with excellent glass-forming ability, thermal stability and unusual pronounced β-relaxation behaviour among known MGs [34] , [35] , is chosen as a model system. Plausible correlations among relaxation behaviours, dynamic heterogeneity, microscopic hidden inhomogeneous flow to macroscopic large-scale homogeneous flow during GLT transition and mechanical behaviours of MGs are established and interpreted by the energy landscape theory. The hidden flow and temperature-dependent tensile experiments It is known that the flow phenomenon in MG is the percolation of the localized flow units [12] , [14] , [21] . To detect the extreme slow hidden flow before yielding or microscopic structural evolution during GLT, we applied Dynamical Mechanical Spectrum (DMS) measurement, which is a sensitive method to detect the viscoelastic properties of MGs [34] , [35] , [36] . The temperature dependence of the loss modulus E ′′ measured at 1 Hz is shown in Fig. 1a . Besides dominant α-relaxation peak at T α =481 K, a β-relaxation peak at T β =363 K can be clearly seen. We note that the definition of T β and T α is frequency dependent. Slowest boundary frequency of 0.01 Hz for both β- and α-relaxation peaks corresponds to an experimental observing time of ~100 s, which is defined as the separation time between glass and liquid [2] , [9] , and definition is helpful for comparison among different glassy systems. The blue and the red regions in Fig. 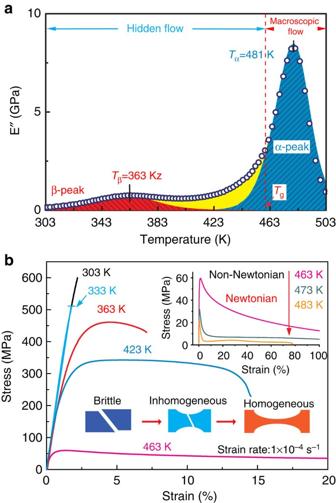Figure 1: Hidden microscopic and macroscopic flow regions in temperature domain. (a) Temperature-dependent loss modulusE′′ (dark blue circles) of La60Ni15Al25MG measured at 1 Hz. The blue region represents the KWW fitting of α-relaxation while the red region represents the fitting of β-relaxation and the yellow region represents the cooperative interaction area. (b) The engineering stress–strain curves (coloured lines) of quasi-static tensile experiments at several representative temperatures from 303 to 463 K. Inset: non-Newtonian to Newtonian flow transition coupled with viscosity change aboveTg. 1a , respectively, represent the fit of α- and β-relaxations by Kohlrausch–Williams–Watts (KWW) equation [21] (The fitting parameters and corresponding storage modulus fitting results can be seen in Supplementary Table 1 and Supplementary Fig. 1 ). The β-relaxation correlates with localized flow unit regions, and its peak intensity in DMS indicates the fraction of flow units in glasses [21] . The unusual pronounced β-relaxation peak in DMS for the La-based MG indicates that the nano-scale localized flow behavior occurs even much below the T g , and the gap area between the α and β peaks implied that cooperative interaction occurs [8] , [37] . Figure 1: Hidden microscopic and macroscopic flow regions in temperature domain. ( a ) Temperature-dependent loss modulus E ′′ (dark blue circles) of La 60 Ni 15 Al 25 MG measured at 1 Hz. The blue region represents the KWW fitting of α-relaxation while the red region represents the fitting of β-relaxation and the yellow region represents the cooperative interaction area. ( b ) The engineering stress–strain curves (coloured lines) of quasi-static tensile experiments at several representative temperatures from 303 to 463 K. Inset: non-Newtonian to Newtonian flow transition coupled with viscosity change above T g . Full size image Figure 1b shows temperature-dependent macroscopic flow phenomena induced by tensile stress. Near room temperature, the MG shows large apparent elastic deformation (~2%) and abruptly breaks when the stress reaches the yield strength value; when the temperature increases to 333 K the MG still shows the pure elastic behaviour, but the fracture strength obviously decreases. By further increasing the temperature, a conspicuous transition from brittle to plastic deformation occurs. Such transition is ascribed to the gradual appearance of multiply shear bands [14] , [38] , [39] , [40] , which stem from unstable localized regions [39] , [41] . A homogeneous flowing deformation with superplasticity over 100% deformation is achieved around T g =461 K under a normal strain rate of 1 × 10 −4 s −1 . When temperature is higher than T g , the apparent macroscopic flow is dominated by viscosity and undergoes the viscous non-Newtonian flow to dilute Newtonian flow transformation [14] , [42] . However, the macroscopic tensile experiments cannot reflect the microstructural changes or microscopic slow flow before the yielding or T g . 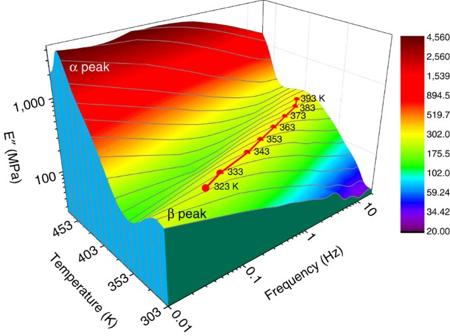Figure 2: Three-dimensional loss modulusE′′ maps with increasing temperature. Results cover 0.01–16 Hz isothermal measured from 303 to 473 K with a temperature step of 10 K. Colours changing from cold blue to warm red represent low to high modulus value.E′′ curve measured at one temperature is marked as thin black line. Every β-relaxation peak is labelled as red dots. Dynamical mechanical relaxation measurements Figure 2 presents the DMS isothermally measured in frequency domain at various temperatures of MG in a three-dimensional form. In frequency domain, at each temperature, we can get DMS for La-based MG to distinguish the α- and β-relaxations within our measuring frequency range (0.01–16 Hz), and the DMS can be obtained from cross-section along the temperature coordinate (indicated as the dark green section in Fig. 2 ). The change of the β-relaxation peak on temperature reflects the evolution of the flow units approaching T g . Both the frequency or temperature-dependent DMS of the MG can be fit by KWW, and the KWW fitting distribution coefficient β is 0.5, which represents the dynamic and structural heterogeneities and can be obtained for either α- or β-relaxations peaks from isochronal and isothermal DMS in Fig. 1a and Fig. 2 (fitting parameters and curves see Supplementary Table 1 and Supplementary Figs 1 and 2 ). The strength ratio between the two relaxation peaks is ~7% from either DMS method. Figure 2: Three-dimensional loss modulus E ′′ maps with increasing temperature. Results cover 0.01–16 Hz isothermal measured from 303 to 473 K with a temperature step of 10 K. Colours changing from cold blue to warm red represent low to high modulus value. E ′′ curve measured at one temperature is marked as thin black line. Every β-relaxation peak is labelled as red dots. Full size image The β-relaxation peaks change and shift in comparison to α-relaxation peaks are indicated in Fig. 2 . The β-relaxation peaks in frequency domain at different temperatures reflect the characteristics and fraction of exact portion suffering GLT transition. Initially, only a part of the flow units is activated at room temperature and no obvious relaxation peak is observed. When the temperature exceeds, more flow units with high activation energy are gradually activated, and the β-relaxation peak appears at ~323 K and then the flow units are fully activated above T β . With increasing temperature, the α- and β-relaxations gradually merge together, the activated flow units percolate and the GLT occurs. It is clear that those flow units reflected by β-relaxation, mainly contribute to the hidden flow at low temperature. Stress relaxation spectra measurements Stress relaxation measurement, which is another powerful tool to reveal the time-dependent liquid-like nature of flow units in MGs [43] , [44] , is applied to study the structural evolution during GLT process. 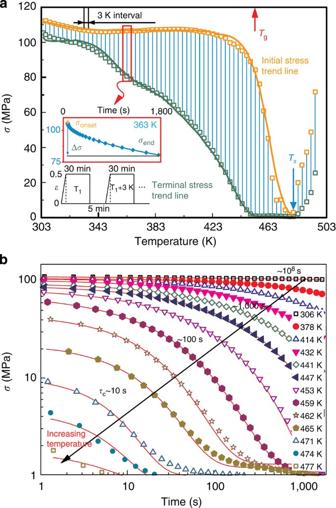Figure 3: Stress relaxation spectra of hidden flow. (a) ‘Harp’-like stress relaxation spectra containing 65 stress relaxation curves (blue line) measured at stepping temperature from 303 to 495 K. Initial stressσonset(orange open block) andσend(dark green open block) trend lines with temperature are deduced from our model. Inset: one enlarged typical stress relaxation curve measured at 363 K. (b) Representative stress relaxation (coloured symbols) and corresponding KWW fitting (red thin lines) curves measured at the temperature range 306–477 K. The log–log plot is adopted for better identification of GLT transition with temperature. Typical order ofτcvalues at different temperatures are marked in figure and exact number can be found inSupplementary Fig. 3. Figure 3a is a stress relaxation spectra containing 65 isothermal stress relaxation curves measured from room temperature beyond T g at a temperature interval of 3 K (for details see the methods section). A typical stress relaxation curve measured at 363 K is shown as inset, where the stress needed to maintain constant strain gradually relaxes with increasing time. Initial stress σ onset and terminal stress σ end can reflect the viscoelastic properties of sample [43] . The lower σ onset value or the larger stress drop Δ σ = σ onset − σ end indicates the larger fraction of liquid-like activated flow units or the smaller viscosity of MG [43] . The shape of stress relaxation curve showing non-exponential behaviour is related with dynamic heterogeneity. The σ onset and σ end of each relaxation curve are enlarged as orange and green open circles, respectively. Decay of the σ end accelerates above T β , whereas the change of σ onset is not prominent until close to T g . The σ end drops to almost zero near T g , while σ onset vanishes at temperature higher than T α . When temperature is higher than T α , the rebirth of stress is due to the disturbance of the occurrence of the crystallization. Figure 3: Stress relaxation spectra of hidden flow. ( a ) ‘Harp’-like stress relaxation spectra containing 65 stress relaxation curves (blue line) measured at stepping temperature from 303 to 495 K. Initial stress σ onset (orange open block) and σ end (dark green open block) trend lines with temperature are deduced from our model. Inset: one enlarged typical stress relaxation curve measured at 363 K. ( b ) Representative stress relaxation (coloured symbols) and corresponding KWW fitting (red thin lines) curves measured at the temperature range 306–477 K. The log–log plot is adopted for better identification of GLT transition with temperature. Typical order of τ c values at different temperatures are marked in figure and exact number can be found in Supplementary Fig. 3 . Full size image Figure 3b highlights several representative stress relaxation curves at different temperatures to investigate characteristic change with temperature. Each curve is rescaled to its measurement time with σ onset at t =0. A log–log plot is adopted here for better identification approaching glass transition. At room temperature, the stress drop is feeble but occurs within our experimental time, this demonstrates that there exist unstable flow unit regions in the MG, even though it looks like an elastic body at low temperature by conventional detection. When the temperature exceeds, the drop of stress starts from the long experimental time tail and gradually accelerates. Above 459 K (close to T g =461 K), the σ end drops to <1 MPa as shown in Fig. 3a , indicating that the whole sample enters into macroscopic flow within an experimental time of ~10 3 s. The stress change with time of all curves can be fitted by KWW-type formula where σ 0 is the initial stress normally equal to σ onset , σ r is the residual stress at infinite time, τ c is the critical stress relaxation time and β KWW is a non-exponential parameter related with dynamic heterogeneity. As glass can be regarded as a frozen liquid with considerable long relaxation time [10] , no pronounced residual stress should be abided at infinite time. Therefore, σ r =0 is taken below 459 K for accurate comparison of fitting parameters (see Fig. 4a and Supplementary Fig. 3 ). All fitting curves are drawn in the figure and some typical values of τ c , over 10 7 orders change during the process, are also shown. 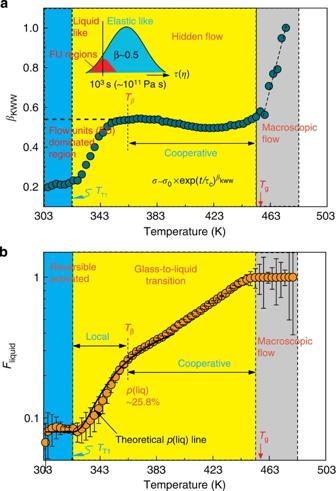Figure 4: The evolution of structure and flow units during hidden flow. (a) Temperature-dependentβKWWvalues (dark green circles) used for fitting stress relaxation curves. Inset: schematic diagram illustrates the separation between liquid-like and elastic-like regions in this study. (b) Evolution path of fraction of liquid-like zonesFliquid(orange circles) with increasing temperature. Three distinct stages separated byTT1andTgare observed during the GLT process. Black line is the theoretical simulating result. AtTβ,Fliquidreaches a connective percolation threshold of 0.25 and isolated-to-cooperative activation transition occurs. Figure 4: The evolution of structure and flow units during hidden flow. ( a ) Temperature-dependent β KWW values (dark green circles) used for fitting stress relaxation curves. Inset: schematic diagram illustrates the separation between liquid-like and elastic-like regions in this study. ( b ) Evolution path of fraction of liquid-like zones F liquid (orange circles) with increasing temperature. Three distinct stages separated by T T1 and T g are observed during the GLT process. Black line is the theoretical simulating result. At T β , F liquid reaches a connective percolation threshold of 0.25 and isolated-to-cooperative activation transition occurs. Full size image We note that the definition of liquid-like or elastic-like strongly depends on observing time [9] . Here the experimental time of each stress relaxation test is elaborately selected at an order of 10 3 s, which corresponds to a critical viscosity value of about 10 11 Pa s at T g for this MG system [45] , [46] . Therefore, portions that perform viscoelastic properties within our experimental time will be treated as liquid-like, otherwise as elastic-like, as illustrated in the inset of Fig. 4a . Based on the KWW fitting of stress relaxation curves, the changes of distribution coefficient β KWW can be obtained and are shown in Fig. 4a . As β KWW is related with the dynamic heterogeneity, smaller β KWW normally indicates wider dynamic heterogeneity distribution of system, and vice versa [45] , [46] , [47] , [48] . Three stages during the evolution can be observed below T g from the temperature-dependent curve of the β KWW . Below 323 K (termed as T T1 ), the β KWW is ~0.2 and remains almost constant. It rapidly increases to 0.55 at T β . After this, its value only slightly changes around 0.5 between T β and T g . As the system relaxation time distribution β =0.5, the value of β KWW should be 0.5 when the sample can be treated as an integral acting like a liquid in a sufficient long time and contributes to the stress decay. However, the viscoelastic property is dominated by those flow units at low temperature as shown in Fig. 2 , and the smaller β KWW below T β should be ascribed to the inhomogeneous activation of flow units. Only isolated, stochastic and reversible flow units can be activated below T T1 . This conclusion can be further verified by fitting of the stress relaxation curve based on the nature of flow units (for details see Supplementary Methods and Supplementary Fig. 4 ). Above T β , an almost constant β KWW around 0.5 indicates that the majority of flow units in the sample start to cooperate with each other and involve in a stress relaxation process at a long but finite time scale. The rapid increase of β KWW above T g is attributed to the exceeding of experimental time when compared with the time needed to attain equilibrium, as represented in Fig. 3b , rather than signifying the homogeneity of the supercooled liquid. The measured stress drop Δ σ = σ onset − σ end reflects the fraction of liquid-like zones [43] , [49] . From Fig. 3a,b , the increase of temperature leads to an increment of Δ σ , indicating that more fractions of atoms in the MG undergo inelastic deformation and are transformed into liquid-like state [50] , [51] . Therefore, we model the MG into two parts: liquid-like zones and elastic matrix. Liquid-like zones are simplified as a distribution of dashpots following the Newtonian law, while elastic matrix are treated as springs with ideal elastic modulus E following Hooke’s law. The fraction of liquid-like zones F liquid and elastic matrix F elastic can be deduced from the σ onset and σ end of each stress relaxation test by and where F liquid +F elastic =1, σ elastic = Eε and . The σ liquid can be estimated based on viscosity relation [10] , [52] and E , ε and are temperature-independent constant values (see Supplementary Methods and Supplementary Fig. 5 ). Figure 4b presents the change of F liquid values with temperature, which shows the similar changing tendency of the distribution coefficient β KWW . Two transition temperatures T T1 and T g are also observed and separate the evolution of F liquid into three regions. From room temperature to T T1 , the F liquid values remain almost constant, indicating that in this region the activation process is reversible and no notable elongation is observed after each stress relaxation test (see Supplementary Fig. 6 ). When temperature is higher than T T1 , more flow units are transformed into liquid state and the MG shows viscoelastic behavior. The F liquid growth rate change or the flow phenomenon becomes noticeable around T β , related with the previous assumption of the isolated-to-cooperative deformations transition. The MG transfers into macroscopic flowing state at T g with fully activated of liquid-like zones and F liquid approaches 1. The changing tendency of F liquid , showing a nonlinear relationship with temperature, further demonstrates a crucial role of the activation of the liquid-like zones in flow and properties of MGs. The equation based on topological fluctuations in the bonding network [53] can also fit our results. The simulation details can be found in Supplementary Methods . The atoms with local volume strain exceeding 0.11 are defined as liquid-like in the theory of ref. 53 . Obviously, our definition from time distribution is broader than the atomic level volume strain distribution. With a latent flow unit fraction of 8%, the theoretical curve fits the evolutionary trend of liquid-like zones well at the range from room temperature to T β , as shown by black line in Fig. 4b . This indicates that the F liquid obtained from a simple mechanical model, can also reflect intrinsic microscopic structural properties of MG. Furthermore, the F liquid reaches a classical percolation threshold between 0.2–0.3 (refs 53 , 54 ) at T β , suggesting that the activated liquid-like zones are no longer isolated above T β . The appearance of these extensive and cooperative flowing spots trigger the brittle-to-ductile mechanical transition. Based on the above results, intrinsic correlations between evolution of flow units, deformation and relaxation maps can be established and can be interpreted by the energy landscape theory. Below T T1 , only reversible flow units can be activated, as illustrated by the high mobility atoms (red balls) embedded in the elastic shell (blue balls) in Fig. 5 . The flow units with high concentration region of free volume may be related with high density inhomogeneity [55] . The fraction of the flow units is ~8% for this specific MG system. Such isolated reversible motions within matrix can be regarded as hopping events across inherent structures and contribute to the β-relaxation [26] , [56] . These few easy flowing spots do not change the brittle nature of MGs. When the temperature continuous to exceed, adjacent weak-bonded regions around flow unit regions are also gradually transformed into liquid state, as the applied strain lowers the energy barrier between adjacent megabasins in energy landscape [51] , [57] , [58] and increase the fraction of the flow units as illustrated in Fig. 5 . At this stage, the liquid-like zones lead to localized plastic events and lower the yielding stress, but the MG shows no macroscopic plasticity. 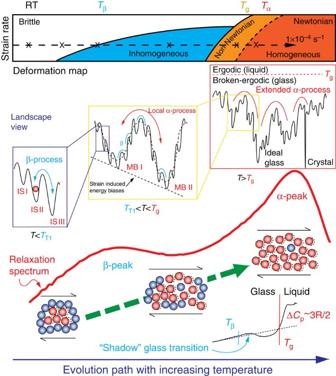Figure 5: Correlation map during hidden flow. Correlations between evolution of liquid-like zones, deformation map, relaxation spectrum and energy landscape are established during glass-to-liquid transition. Figure 5: Correlation map during hidden flow. Correlations between evolution of liquid-like zones, deformation map, relaxation spectrum and energy landscape are established during glass-to-liquid transition. Full size image Around T β , a connectivity percolation of liquid-like zones occurs. The percolation of the flow units forms the multiply shear bands [59] , leading to ductile deformation [21] , [25] . For most MGs, T β is located at about 0.8–0.9 T g (refs 35 , 60 ), which is close to homogeneous deformation boundary at 0.9 T g in deformation map [14] . Higher strain rate should correspond to a faster boundary frequency and a higher fully activated β-relaxation temperature T β ′ , and vice versa . Another arresting phenomenon around T β is the sub- T g endothermic peak or termed shadow glass transition in glasses [61] , [62] . This endothermic peak is thought to be related with β-relaxation but the intuitive physical picture is still not clear [61] . From our scenario, cooperative translational movements [35] , [63] take place above T β and can be regarded as a kind of confined GLT, leading to an endothermic peak. Such hidden flowing movements need external energy to facilitate. This also explains the reason that the endothermic peak is always slightly higher than the T β measured by dynamical method, because additional mechanical disturbance is needed to motivate the cooperative flow events. Meanwhile, the slower growth rate of F liquid also originates from the cooperative movements, as the activation energy of cooperative α-relaxation is three times larger than isolated β-process (see Supplementary Fig. 7 ). When temperature approaches T g , the sample behaves macroscopic flowing under our observing time. A heat capacity jump of about 3R/2 related to translational freedom addition [64] can be observed and a critical transition from broken-ergodic to ergodic on energy landscape occurs. The sample transforms into liquid-like above T g , the viscosity change becomes the dominating factor for the deformation behaviours. As viscosity rapidly decreases and approaches T α , the sample transitions from non-Newtonian to Newtonian flow as marked in the deformation map of Fig. 5 . In summary, a panorama picture revealing the evolution of localized flow from low temperature glassy state to supercooled liquid state is offered to understand the deformation and relaxation maps and the GLT. Unstable flow units are demonstrated to persist in glassy state and their reversible activation contributes to the viscoelasticity. These liquid-like zones show a nonlinear increase with temperature and their properties play a crucial role in determining diverse flow phenomena in glasses. A connective percolation state is achieved above T β and leads to the ductile deformation and a cooperative GLT process. Our results might shed light on the mechanism of flowing phenomena in glassy state and provide a practical guideline in controlling mechanical behaviour in MGs. Sample preparation Ribbons and bulk La 60 Ni 15 Al 25 MG were prepared by melt-spinning and Cu-mold casting methods in argon atmosphere, respectively. The thickness of the ribbons are about 40 μm and the diameter of the MG rods are 2 mm. The glass transition temperature of the La 60 Ni 15 Al 25 samples is located at 461 K. The tensile mechanical tests and stress relaxation measurements were performed with ribbons, while DMS results are obtained with rods. The conclusion obtained in the tension and the evolution trends is the same for both as thin ribbons and bulk sample form. Structural and dynamic characterization The glassy nature of the samples was ascertained by X-ray diffraction (a MAC Mo3 XHF diffractometer with Cu Kα radiation). The differential scanning calometer (DSC) measurements were conducted by using a Perkin-Elmer DSC-7 at a heating rate of 20 K min −1 (see Supplementary Fig. 8 ). Dynamical mechanical behaviour was measured using temperature ramp mode and frequency sweep mode on a TA DMA Q800. Under temperature ramp mode, the sample was measured at a heating rate of 3 K min −1 and only 1 Hz results were shown here. Meanwhile, frequencies covering 0.01–16 Hz were used with a temperature step of 10 K in frequency sweep mode. Uniaxial tensile tests of MG ribbons were carried out over a temperature range (303–483 K) under 1 × 10 −4 s −1 in the same dynamical mechanical analyzer machine. Stress relaxation measurements Measurements were performed on TA DMA Q800 and ribbon samples were mounted in tension clamp. A constant strain of 0.5% was rapidly applied on the sample and held for 30 min for each test to record the stress decay. The stress relaxation measurements for the same sample were tested from 303 to 495 K (> T g ) with a step of 3 K, and a total of 65 stress relaxation tests were conducted. The interval between the adjacent two tests is 5 min, including a 3-min isothermal holding time at the next measured temperature to avoid thermal fluctuations. Besides, to assure the accuracy of the strain value, the length of sample was measured before and after each stress relaxation test. How to cite this article: Wang, Z. et al. Evolution of hidden localized flow during glass-to-liquid transition in metallic glass. Nat. Commun. 5:5823 doi: 10.1038/ncomms6823 (2014).